Layer-by-layer assembly of vertically conducting graphene devices Graphene has various potential applications owing to its unique electronic, optical, mechanical and chemical properties, which are primarily based on its two-dimensional nature. Graphene-based vertical devices can extend the investigations and potential applications range to three dimensions, while interfacial properties are crucial for the function and performance of such graphene vertical devices. Here we report a general method to construct graphene vertical devices with controllable functions via choosing different interfaces between graphene and other materials. Two types of vertically conducting devices are demonstrated: graphene stacks sandwiched between two Au micro-strips, and between two Co layers. The Au|graphene|Au junctions exhibit large magnetoresistance with ratios up to 400% at room temperature, which have potential applications in magnetic field sensors. The Co|graphene|Co junctions display a robust spin valve effect at room temperature. The layer-by-layer assembly of graphene offers a new route for graphene vertical structures. Graphene, comprising one monolayer of carbon atoms packed into a two-dimensional (2D) honeycomb lattice, has received great attention due to its unique properties, including massless Dirac fermions, a linear dispersion relation near the Dirac cones, high carrier mobility, emerged quantum confinements and gate-tunable optical transitions [1] , [2] , [3] , [4] , [5] , [6] , [7] . In addition, with very long spin-flip time [8] and weak spin-orbit coupling [9] , graphene has been proposed as an ideal material for spintronics. High-yield production and large-area synthesis of graphene have been achieved, which facilitate its use in transparent electrodes, interconnections and wafer-scale electronics [10] , [11] , [12] , [13] , [14] , [15] . Nevertheless, both fundamental and application-oriented graphene investigations are commonly concerned with the graphene 2D plane. Recently, graphene-based vertical devices have raised considerable interest [16] , [17] , [18] . Field-effect tunnelling transistors based on vertical graphene|insulating barrier|graphene heterostructures [17] and a gate-controlled Schottky barrier based on graphene|silicon heterostructures [18] , were demonstrated to achieve large current switching ratios. Graphene|Al 2 O 3 |graphene heterostructures were studied to probe the Coulomb drag of massless fermions in graphene [19] . For graphene|semiconductor and graphene|dielectric vertical devices, thermionic emission or tunnelling effects dominate the transport properties. However, few studies focus on graphene|metal vertical transport devices. Without tunnelling or Schottky barriers, graphene|metal devices have high conductivity and may have potential applications in conductive electrodes, sensors and spintronics. The graphene|metal and graphene|graphene interfaces have an important role in graphene vertically conducting devices. Therefore, it is highly desirable to gain a deep understanding of the graphene interface properties and exploit new functional devices. Here we develop a general method to construct graphene vertical devices with controllable functions via choosing different interfaces between graphene and other materials. Vertically conducting magnetic field sensors and spin valves are demonstrated, via bottom-up fabrication of the Au|graphene|Au and Co|graphene|Co structures, respectively. The importance of the interface is revealed through systematic magneto-transport measurements at both low temperature and room temperature. Au|graphene|Au devices with deposited top electrodes The sketch of Au|graphene|Au device is shown Fig. 1a . The device fabrication processes are briefly described as follows. First, the bottom electrodes are fabricated using electron beam lithography (EBL), followed by metal deposition of Ti/Au (5/25 nm) and lift-off. Second, we can transfer the monolayer graphene using poly(methyl methacrylate) (PMMA) microstamp onto the bottom electrode [20] . After removing the PMMA on graphene, another layer of graphene can be stacked ( Supplementary Fig. S1 ). Via layer-by-layer transfer of the monolayer graphene, the layers of the graphene stack can be controlled. The multilayer graphene stacks show similar Raman spectrum features to monolayer graphene ( Supplementary Fig. S2 ). The third step is to fabricate the top electrode by another round of EBL and metal deposition of Au (50 nm) via electron-beam evaporation. A four-terminal cross bar configuration was adopted to perform the measurement of the vertically conducting device, as illustrated in Fig. 1a . A constant current source was connected to one arm of the bottom electrode and one arm of the top electrode, and the other pair of leads was used to measure the voltage drop. The reliability of the four-probe measurement was verified, because no voltage drop was measured when testing the cross-bar structure without the graphene layer. 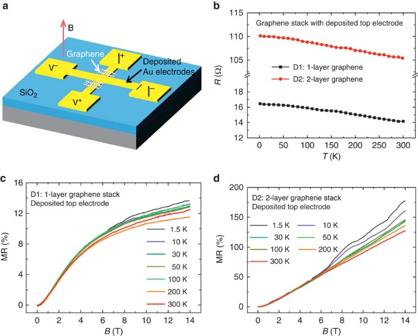Figure 1: Transport properties of vertically conducting Au|graphene|Au with deposited top Au electrode. (a) Schematic diagram for the Au|graphene|Au junction, where the top Au electrode was fabricated via the processes including EBL, metal deposition and lift-off. (b) Resistance as a function of temperature for a monolayer graphene (labelled as D1) and a two-layer graphene (labelled as D2) stacks. (c,d) The MR of (c) D1, and (d) D2 measured at different temperatures. Figure 1: Transport properties of vertically conducting Au|graphene|Au with deposited top Au electrode. ( a ) Schematic diagram for the Au|graphene|Au junction, where the top Au electrode was fabricated via the processes including EBL, metal deposition and lift-off. ( b ) Resistance as a function of temperature for a monolayer graphene (labelled as D1) and a two-layer graphene (labelled as D2) stacks. ( c , d ) The MR of ( c ) D1, and ( d ) D2 measured at different temperatures. Full size image Figure 1b displays the temperature dependent resistance of monolayer graphene (labelled D1) and a two-layer graphene stack (labelled D2), respectively. A small increase of their resistances is observed as the temperature decreases from 300 to 1.4 K. This is probably due to randomly distributed impurities coming from the impact of metal atoms during the electrode deposition process. The magnetoresistance (MR) was measured by applying the magnetic field perpendicular to the substrate plane. The magnetic field dependent resistances of D1 and D2 are shown in Fig. 1c . For D2, a large positive MR (defined as MR= R ( B )/ R (0)−1) about 180% is observed at 1.4 K under 14 T. In contrast, a much smaller MR about 14% at 14 T with a sign of saturation is observed for D1. For the vertically conducting graphene devices, the carrier transport properties are dominated by the graphene|Au and graphene|graphene interfaces. The metal deposition may cause damage of graphene and produce defects, vacancies and pinholes because of bump from evaporated atoms, which significantly influence the performances of the vertical monolayer graphene device. For sample D1, some parts of the deposited top electrode may directly contact with the bottom electrode through some pinholes in the monolayer graphene, so the graphene was partially shorted and small MR effect was observed. However, for sample D2, the short circuit can be largely avoided. Consequently, the observed large MR in sample D2 may be originated from the Au|graphene or graphene|graphene interfaces. Au|graphene|Au devices with transferred top electrodes To further reveal the origin of the large MR, we fabricated the graphene stack devices by transferring the top metal electrode instead of depositing the top Au electrode for comparison. The top electrode was fabricated by transferring a gold strip (100 nm in thickness) onto the graphene stacks with just same technique as used for the graphene transfer ( Supplementary Fig. S3 ). An optical image of a typical device and the measurement configuration are shown in Fig. 2a . 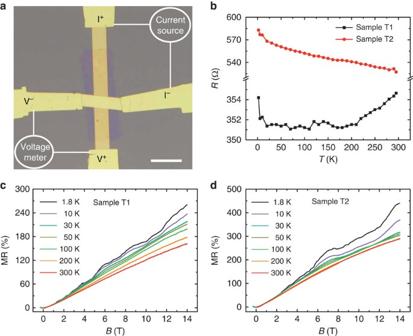Figure 2: MR of graphene stacks with transferred top Au electrode. (a) Optical image and sketch of measurement configuration of a graphene vertically conducting device. Scale bar, 20 μm. (b) R–T behaviours for a monolayer graphene (sample T1) and a two-layer graphene stack (T2). (c,d) The MR of (c) T1, and (d) T2 measured at different temperatures. Figure 2: MR of graphene stacks with transferred top Au electrode. ( a ) Optical image and sketch of measurement configuration of a graphene vertically conducting device. Scale bar, 20 μm. ( b ) R–T behaviours for a monolayer graphene (sample T1) and a two-layer graphene stack (T2). ( c , d ) The MR of ( c ) T1, and ( d ) T2 measured at different temperatures. Full size image Figure 2b shows R(T) of a monolayer graphene (labelled T1) and a two-layer graphene stack (labelled T2) with a transferred Au electrode. The resistances show weak temperature dependence, suggesting the graphene is of high quality [21] . Figure 2c present the MR of T1 and T2 at different temperatures with the magnetic field perpendicular to the graphene plane. It is surprising that a very large positive MRs of 260 and 440% at 14 T and 1.8 K for T1 and T2 was observed, respectively. Moreover, the MR effect is still tremendous at 300 K, 160% and 250% at 14 T for T1 and T2, respectively. One can see from Fig. 2c that the MR shows weak temperature dependence below 2 T and there is no sign of saturation up to 14 T. Nevertheless, the MR effect is rather small when the magnetic field is parallel to the graphene plane ( Supplementary Fig. S4 ). Our experimental results demonstrated that the perpendicular magnetic field can notably affect the carrier transport, suggesting that the carrier transport through graphene must have an in-plane velocity component, which is perpendicular to direction of the magnetic field. The in-plane carrier velocity may be due to the existence of wrinkles in the transferred graphene, which was further confirmed by the atomic force microscope image ( Supplementary Fig. S5 ). As the transferred top Au electrode was paved on the wrinkled graphene, the carriers have to move along the graphene slope from the top electrode to the bottom electrode, resulting in the in-plane velocity component. Owing to the low resistance of the devices, the vertical carrier transport may be dominated at zero magnetic field. Nevertheless, the in-plane carrier transport may be responsible for the observed MR as the magnetic field was applied perpendicular to the substrate. Similar linear MR has also been observed in many systems, such as multilayer epitaxial graphene [22] , single-crystal InSb and polycrystalline InSb [23] . The linear MR has two prevailing models: the quantum model [24] , [25] and the classical model [26] . The quantum linear model requires that the Landau levels are well formed (μB>1) and all electrons coalesce into the lowest Landau level at low temperatures. However, the large MR in our devices persists up to room temperature and has weak temperature dependence. So the quantum model may be not a suitable explanation for our experiments. Parish and Littlewood [26] , [27] suggested a classical description for linear MR in a strongly inhomogeneous system arising from the fluctuations in the carrier mobility. For our samples, the atomic force microscope measurements show that the transferred graphene layers are largely inhomogeneous, and there are two types of carriers in graphene resulting in inhomogeneous spatial distribution of the carrier mobility. Therefore, our observed large MR may be attributed to the Parish and Littlewood theory. Quantum transport in Au|graphene|Au devices As shown in Fig. 2a , except the graphene sandwiched between two electrodes, partial graphene sheet directly lays on the SiO 2 substrate. The carrier density of the graphene outside of the electrode area (laying on SiO 2 substrate) can be tuned by applying a back gate voltage. The carrier diffusion can occur between the graphene regions inside and outside of the electrode area to reach a new balance, and thus the carrier density of the graphene inside of the electrode area can also be tuned by the gate voltage. As shown in Fig. 3 , the resistances of the samples T1 ( Fig. 3a ) and T2 ( Fig. 3c ) can be efficiently modulated by the gate voltage using the Si substrate as the back gate electrode and the bottom/top Au electrodes as the source/drain electrodes. At zero magnetic field, it is noting that the R–V g curves are smooth at high temperatures while display oscillations at low temperatures, as shown in Fig. 3a . The resistance oscillations at 1.8 K and 0 T are more notable through subtracting the background ( Supplementary Fig. S6 ). As the spacing between the top/bottom electrodes is comparable with the Fermi wavelength ( λ f ) of the carriers in graphene, where is tunable by changing the carrier concentration n s by applying gate voltage ( V g ), here g s , g v are spin degeneracy and valley degeneracy, respectively. The Au|graphene|Au structure can be considered as a Fabry–Perot cavity for electron waves. On the other hand, universal conductance fluctuations may also be notable at low temperatures. The observed quantum oscillations are ascribed to the quantum interference effect in Au|graphene|Au heterostructures. 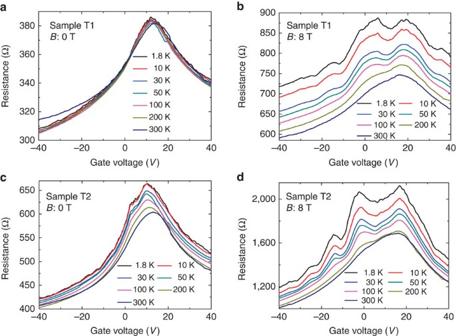Figure 3: Gate voltage tunable transport properties. (a,b) Resistance versus gate voltage (R–Vg) of sample T1 at different temperatures and (a) at zero magnetic field, (b) under 8 T. (c,d) TheR–Vgcurves of sample T2 at different temperatures and (c) at zero magnetic field, (d) under 8 T. Figure 3: Gate voltage tunable transport properties. ( a , b ) Resistance versus gate voltage ( R – V g ) of sample T1 at different temperatures and ( a ) at zero magnetic field, ( b ) under 8 T. ( c , d ) The R – V g curves of sample T2 at different temperatures and ( c ) at zero magnetic field, ( d ) under 8 T. Full size image The transport properties are also influenced by the quantized Landau levels in graphene under high magnetic field. As shown in Fig. 3b , under 8 T, the large peaks in resistance are corresponding to the carriers filling of the Landau levels controlled by gate voltage. The large peaks/valleys gradually disappear with increasing temperature, which are consistent with the Shubnikov-de Haas (SdH) oscillations. The observation of SdH oscillations further confirms that the carriers have in-plane velocity component in graphene. Au|graphene|Au devices with minimum PMMA residue It has been reported that there may have PMMA remains on graphene during transfer process. To reveal how the PMMA remains influence the vertical transport properties, current–voltage (I–V) curves of a typical Au|graphene|Au device with transferred top electrode were measured. Here, the PMMA on graphene was removed by acetone. Surprisingly, the device displays linear I–V curves at both 300 and 1.8 K ( Supplementary Fig. S7 ), indicating the good ohmic contacts between the electrode and graphene. To reveal the underlying mechanism, the graphene surface was further studied by high-resolution field emission SEM. For the graphene with PMMA removed by acetone, the PMMA residues cover the graphene with many narrow pinholes with width of ~60 nm ( Supplementary Fig. S8a ). Therefore, the dominated transport takes place through the narrow pinholes, resulting in the metallic contact and linear I–V curves. The PMMA residues only reduce the graphene/metal contact area and increase the device resistance. In order to further remove the PMMA residues on graphene, the monolayer graphene transferred on the Au electrode was annealed at 350 °C for 3 h in the gas flow of 20 sccm H 2 and 100 sccm Ar. After annealing the PMMA residues are effectively reduced ( Supplementary Fig. S8b ). 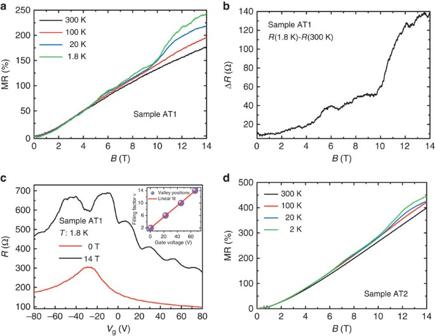Figure 4: MR of Au|graphene|Au stacks with minimum PMMA residue after annealing. (a) The MR of an Au|monolayer graphene|Au device (sample AT1). The top electrode was fabricated via transferring a gold strip after the PMMA residues on graphene were reduced by annealing. (b) The resistance difference between 1.8 and 300 K (R(1.8 K)−R(300 K)) of sample AT1 shows the deviation from linear magnetic field dependence and the appearance of oscillations at high magnetic field. (c) The SdH oscillations of sample AT1 under 14 T as a function of carrier concentration tuned by back gate voltage. Inset: the filling factor of the SdH oscillations as a function of the valley position in gate voltage. (d) The MR of an Au|two-layer graphene|Au device without any PMMA residues between the graphene layers (sample AT2). Figure 4a shows the MR of the annealed monolayer graphene (labelled AT1) with a transferred Au electrode. Positive linear MR of ~175% at 14 T was observed at 300 K. At low temperatures and under high magnetic field, the quantized Landau levels make the MR departing from linear dependence and the appearance of oscillations, as shown Fig. 4b . The SdH oscillations were demonstrated more clearly under 14 T via tuning the carrier concentration by back gate voltage, as shown in Fig. 4c . The valley positions of the resistance oscillations show a linear dependence with the Landau filling factor ν = g s g v ( N +1/2), where N = n s ( h / g s g v e )(1/ B ) is an integer, h is Planck’s constant, g s =2 and g v =2. At 14 T, the Δ n s and Δ V g between two neighbour Landau levels is 1.35 × 10 12 cm −2 and 22 V, respectively. The tunability of 6 × 10 10 cm −2 V −1 is well consistent with the linear tunability of graphene carrier concentration via 285 nm SiO 2 dielectric layer. Figure 4: MR of Au|graphene|Au stacks with minimum PMMA residue after annealing. ( a ) The MR of an Au|monolayer graphene|Au device (sample AT1). The top electrode was fabricated via transferring a gold strip after the PMMA residues on graphene were reduced by annealing. ( b ) The resistance difference between 1.8 and 300 K ( R (1.8 K)− R (300 K)) of sample AT1 shows the deviation from linear magnetic field dependence and the appearance of oscillations at high magnetic field. ( c ) The SdH oscillations of sample AT1 under 14 T as a function of carrier concentration tuned by back gate voltage. Inset: the filling factor of the SdH oscillations as a function of the valley position in gate voltage. ( d ) The MR of an Au|two-layer graphene|Au device without any PMMA residues between the graphene layers (sample AT2). Full size image For the two-layer graphene stack, we developed a new method to obtain a clean interface between graphene layers without involving any PMMA ( Supplementary Fig. S9 ). Briefly, after the first layer of graphene|PMMA film was separated from the Cu foil, another Cu foil with graphene grown on it was used to fish the graphene|PMMA film out from the deionized (DI) water. Thus, a clean interface without any PMMA between graphene layers was obtained. Then the two-layer graphene transferred on the Au electrode was annealed under the same condition as that of the monolayer graphene. This treatment of the interface can strongly improve the device performance. For the Au|two-layer graphene|Au device, the MR was improved to 400% at 300 K with linear magnetic field dependence and no sign of saturation ( Fig. 4d ). Moreover, the MR is almost temperature independent below 5 T under the range from 300 to 2 K. The advanced performances of the Au-graphene-Au stack make it has potential applications on magnetic field sensors. Spin valves based on Co|graphene|Co vertical junctions Motivated by the novel phenomenon of the vertically conducting Au|graphene|Au structure and the theoretical prediction of extremely large spin filtering efficiencies for FM|graphene|FM (FM=Co, Ni) junctions [16] , [28] , we constructed Co|graphene|Co junctions using the fabrication method similar to the Au|graphene|Au devices. Considering that Co electrodes are easily oxidized, the bottom Co electrode was protected by transferring the graphene onto the Co electrode as soon as possible. Usually the exposure time of the bottom Co electrode in the air was less than 3 min. The top Co electrode was deposited on the surface of graphene by e-beam evaporation and the oxidation of Co was prevented by covering a thin layer of gold. The Co|graphene|Co devices demonstrated linear I–V curves ( Supplementary Fig. S10 ), indicating that the dense Co oxidation layer on the bottom electrode may not be formed and Ohmic property is dominant rather than tunnelling effect. The magneto-transport of the spin valves was measured while sweeping in-plane magnetic field and the applied current was 10 μA. 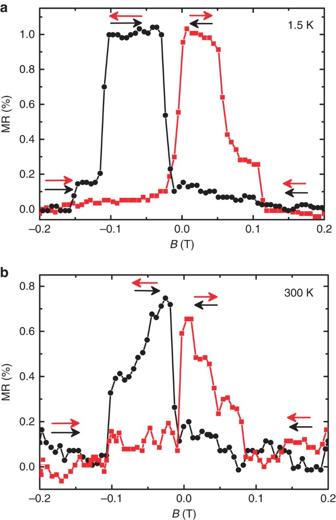Figure 5: Spin valves of Co|graphene|Co vertical structures. The MR of the spin valve based on two-layer graphene stack without any PMMA residues between the graphene layers measured at (a) 1.5 and (b) 300 K, as sweeping the magnetic field parallel to the graphene plane. Figure 5 shows the typical spin valve signals of a Co|two-layer graphene stack|Co device at both 1.5 and 300 K, where the two-layer graphene stack was fabricated without involving any PMMA between the graphene layers ( Supplementary Fig. S9 ). The spin dependent transport through the Co|graphene|Co junction can be described by the MR=[( R AP − R P )/ R P ] × 100%, where R AP and R P are the resistances for the antiparallel and parallel magnetizations of the Co electrodes, respectively. As shown in Fig. 5a , the device is at a low R P state under high magnetic field and changes to a high R AP state as sweeping the magnetic field to opposite direction to inverse the magnetization orientation of one Co electrode. The clear transitions between high resistance state and low resistance state indicate potential application in nonvolatile memories. Figure 5: Spin valves of Co|graphene|Co vertical structures. The MR of the spin valve based on two-layer graphene stack without any PMMA residues between the graphene layers measured at ( a ) 1.5 and ( b ) 300 K, as sweeping the magnetic field parallel to the graphene plane. Full size image For the Co|graphene|Co devices, similar large MR appears under vertical magnetic field as that in Au|graphene|Au device ( Supplementary Fig. S11 ), which further confirms that graphene substantially contributes to the transport in the Co|graphene|Co device. Similar spin valve behaviour of monolayer graphene sandwiched between two Co electrodes was also observed ( Supplementary Fig. S12 ), which suggests that one layer graphene is sufficient enough to uncouple the top and bottom ferromagnetic cobalt layers. In our Co|graphene|Co devices, carrier direct tunnelling from the bottom to top Co electrodes cannot be neglected as there is only one-layer or two-layer graphene stack between them, which is responsible for the observed small MR of the spin valves. The MR of the spin valve can be further improved through adding the number of layers of the graphene stack to suppress the carrier tunnelling between the electrodes. Our developed method of layer-by-layer assembly of graphene provides a route to construct three-dimensionally integrated graphene devices. The graphene microstamps act as building blocks for the bottom-up fabrication of various functional devices. The bottom-up assembly of graphene devices extends the manufacturing strategy from the 2D plane to vertical architecture and provides a new approach for investigating the interactions between assembled graphene layers. In conclusion, we have established a convenient method to construct vertically conducting graphene devices. Magnetic field sensors based on Au|graphene|Au junctions and spin valves based on Co|graphene|Co junctions were demonstrated. Our results reveal the important effect related to the graphene|metal electrode and graphene|graphene interfaces for the grapheme-based vertical devices. The vertical assembly of graphene not only provides a new pathway to explore the electron transport properties but also opens up new vistas of electronic applications. Site-specific transfer-printing of graphene microstamp The monolayer graphene was grown on copper foil by chemical vapour deposition method. The Cu foil with graphene was fixed on a Si substrate. A PMMA thin layer was then spin-coated on the graphene surface. The PMMA|graphene microstamps were patterned via EBL and O 2 plasma etching. A hole with diameter of ~2 μm was formed on each microstamps. The Cu foil was dissolved by FeCl 3 saturated solution for 30 min. The graphene/PMMA film was washed three times by 60 °C DI water. The thin film containing thousands of graphene|PMMA microstamps was then fished out by a metal ring with ~1 cm inner diameter. The graphene|PMMA microstamps were transferred and printed by a micromanipulator with three-axis oil hydraulic controller under an optical microscope. A glass tip with diameter ~500 nm mounted on the micromanipulator was inserted into the hole of the graphene|PMMA microstamp and pulling off the microstamp from the whole membrane. The graphene|PMMA microstamp was then put down on the target position. Fabrication of Au|graphene|Au with deposited top electrode The bottom electrode was fabricated using EBL, followed by metal deposition of Ti/Au (5/25 nm) and lift-off process. We then transferred a graphene|PMMA microstamp onto the bottom Au electrode. The PMMA on graphene was dissolved in acetone. If necessary, another graphene|PMMA stamp was transferred onto the first graphene and then dissolved PMMA in acetone. Third, another round of EBL was employed and the top electrode was fabricated by metal deposition of gold onto the graphene stacks. Raman spectrum characterizations One monolayer graphene|PMMA stamp was transferred and printed on SiO 2 /Si substrate. The PMMA was then dissolved by acetone. The Raman spectrum of the monolayer graphene was measured. Another graphene|PMMA stamp was printed to superpose onto the previous graphene layer. After the PMMA was dissolved by acetone, the Raman spectrum of the two-layer graphene stack was then measured. The Raman spectrum of three-layer graphene stack was also measured after another graphene|PMMA stamp was superposed and dissolving PMMA by acetone. Similarly, the Raman spectrums of four-layer and five-layer graphene stacks were measured. Fabrication of Au|graphene|Au with transferred electrode The bottom electrode and the graphene on the bottom electrode were fabricated using the same transfer-printing method. Using the method similar with the graphene transfer technique, a gold strip was transferred onto the graphene as a top electrode and forming the crossbar configuration. The Au strips were fabricated as follows. Au strips were prefabricated on SiO 2 /Si substrate via EBL and metal deposition. A PMMA thin layer was then spin-coated on the substrate. The PMMA microstamps comprising Au strip were patterned via EBL. The SiO 2 was dissolved by HF solution and the Au-|PMMA-film floated on the solution surface. The Au|PMMA film was then cleaned using DI water. The Au|PMMA film was then fished out by a copper mesh. We then transferred an Au|PMMA microstamp onto the graphene surface as the top electrode. The PMMA on graphene was dissolved in acetone. Fabrication of stacks without PMMA between graphene layers First, a PMMA thin layer was spin-coated on a monolayer graphene surface grown on copper foil. The Cu foil was then dissolved by FeCl 3 saturated solution for 30 min. The graphene|PMMA film was washed three times by 60 o C DI water. Another monolayer graphene on copper foil was used to fish out the graphene|PMMA film from DI water. Because of the face-to-face superposition of graphene layers of the sides with clean surface, there is no any PMMA between the graphene layers. The two-layer graphene|PMMA film was then patterned into microstamps via EBL and O 2 plasma etching. After the Cu foil was dissolved and the two-layer graphene/PMMA film was rinsed, the two-layer graphene|PMMA microstamps can be transferred and printed onto the bottom electrode. Electrical transport measurement The metal|graphene|metal vertically conducting devices were placed in an Oxford cryostat instrument with a variable temperature insert. The temperature ranging from 1.4 to 300 K can be obtained via a temperature controller. The magnetic field can be swept up to 14 T. The electrical signals were measured via low-frequency lock-in techniques. Adopting the four-terminal cross bar configuration, constant current was applied between one lead of the bottom electrode and one lead of the top electrode, and the rest pair of electrode leads was used to measure the voltage drop. How to cite this article: Chen, J.-J. et al . Layer-by-layer assembly of vertically conducting graphene devices. Nat. Commun. 4:1921 doi: 10.1038/ncomms2935 (2013).